Ediacaran 2,500-km-long synchronous deep continental subduction in the West Gondwana Orogen The deeply eroded West Gondwana Orogen is a major continental collision zone that exposes numerous occurrences of deeply subducted rocks, such as eclogites. The position of these eclogites marks the suture zone between colliding cratons, and the age of metamorphism constrains the transition from subduction-dominated tectonics to continental collision and mountain building. Here we investigate the metamorphic conditions and age of high-pressure and ultrahigh-pressure eclogites from Mali, Togo and NE-Brazil and demonstrate that continental subduction occurred within 20 million years over at least a 2,500-km-long section of the orogen during the Ediacaran. We consider this to be the earliest evidence of large-scale deep-continental subduction and consequent appearance of Himalayan-scale mountains in the geological record. The rise and subsequent erosion of such mountains in the Late Ediacaran is perfectly timed to deliver sediments and nutrients that are thought to have been necessary for the subsequent evolution of sustainable life on Earth. In rare cases, the movement of Earth’s crustal plates causes relatively buoyant continental crust to be subducted to high-pressure (HP) and ultrahigh-pressure (UHP) conditions (that is, depth >90 km) and exhumed back to the surface. It has been recently recognized that exhumed UHP rocks derive from subducted continental margins, where the cold and dense slab of oceanic crust pulls the attached continental crust to mantle pressures [1] , [2] , [3] . These HP/UHP rocks are exhumed during the collision that immediately follows subduction of the margin—within 2–30 million years (m.y. )—at rates of mm to cm per year [4] , [5] . UHP crustal rocks appear relatively late in the Earth’s history. The oldest coesite-bearing eclogite is c. 620 Myr old and is found in Mali [6] , [7] , which is part of the West Gondwana Orogen (WGO). However, this has been an isolated finding, and the extent of this deep continental subduction zone and its relation to the development of the orogen remain unknown. If deep subduction and continental collision demarked by the HP/UHP rocks is an orogen-scale feature, it is likely to have had important consequences for the tectonic and environmental evolution of the planet. On modern Earth, the collisional mountain chain that makes the Himalayas is thought to have had profound influence on both climate and tectonics [8] , [9] , [10] , [11] . Despite the occurrence of older and hotter eclogites or high-pressure granulites [12] , [13] , it has been argued that the first appearance of low-temperature/high-pressure rocks during the Neoproterozoic marks the onset of modern plate tectonics dominated by the subduction of very cold slabs [14] , [15] . The lack of such cold geotherms along the subduction channel in the large pre-Neoproterozoic orogens (that is, Grenville Orogen) has been suggested to indicate a different tectonic regime more compatible with shallower and hotter subduction processes [15] . The Neoproterozoic era (1,000–540 Myr), and particularly the Ediacaran period (635–540 Myr), marks a time when life on Earth underwent significant changes with the rise of the metazoans [16] . At the same time, systematic increases of 87 Sr/ 86 Sr in the oceans [17] took place, while the largest known absolute increase in atmospheric p O 2 occurred [18] at c. 600-570 Myr. Major rises in atmospheric p O 2 throughout Earth’s history have been linked to the supply of massive quantities of sediments from mountain belts that were produced during the amalgamation of supercontinents [19] , especially during the Gondwana assembly. The existence of such mountain belts in the Ediacaran and Cambrian periods was postulated based on the chronology of sediments and rare metamorphic rocks [20] , [21] . However, key factors for this model, such as the exact timing and spatial distribution of the change from subduction- to collision-dominated tectonics, and the size of the collisional mountain belt have not yet been constrained. In this article, we investigate the timing and metamorphic conditions of HP/UHP rocks from three key localities distributed along the WGO and compile the magmatic and sedimentary record of this vast collisional zone. We document coincident deep continental subduction along an extensive section of the WGO (at 620-610 Myr) and argue that this marks the onset of the formation of mountain chains that involve continental subduction at mantle depths (that is, UHP metamorphism) with similar magnitude to the Himalayas. We discuss the potential consequences of such large-scale tectonic events for the environmental conditions that underpin the radiation of life in the Ediacaran. The West Gondwana Orogen The Neoproterozoic WGO ( Fig. 1 ) is a linear belt that extended for more than 4,000 km from present-day northeast Africa to Central Brazil [22] , [23] . Modern and traditional views suggest that this orogen resulted from the consumption and closure of the Goiás-Pharusian Ocean [22] , [23] , [24] that culminated in a continent–continent collision involving mainly the conjoined Amazon and West African cratons against the São Francisco-Congo and Saharan cratons ( Fig. 1a ). The rocks involved in this orogen record long-lived, accretionary convergent tectonics since the Early Neoproterozoic with development of several intra-oceanic and continental arcs that are now preserved within a deeply eroded, paleo collisional zone [24] , [25] , [26] , [27] , [28] . The orogen has a protracted tectonic history (over 400 m.y., Fig. 1 ), from the inception of oceanic arc-related juvenile magmatism at c. 850 Myr to terminal continental collision at c. 615–610 Myr, to post-collisional granites and basin infilling at 580–500 Myr. The orogen can be subdivided into four different sectors ( Fig. 1c ) that all have key features that are observed in modern collision zones such as the Alps and the Himalayas. Ophiolites represent remnants of oceanic crust that once separated the continental blocks and they can be found as elongated units within the suture zone, as exemplified by the Bou Azzer ophiolite in Morocco [29] . The dominant rock types between the cratonic blocks are interpreted as passive margin deposits, early (juvenile)- and late-arc-related rock assemblages and syn-orogenic supracrustal sequences. The erosion of mountains that resulted from the collision is documented in post-collisional sedimentary deposits, and the termination of orogenic activity is dated by the age of post-collisional granitoids at c. 580–540 Myr [24] , [27] , [30] . 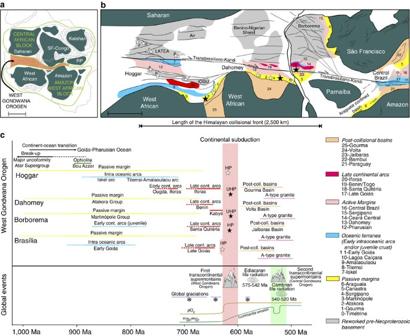Figure 1: Geological context and tectonics of the West Gondwana Orogen. (a) Main cratons and tectonic blocks involved in the formation of the collisional West Gondwana Orogen (scale bar, 1,000 km). (b) Spatial distribution of high-pressure and ultrahigh-pressure rocks and main lithotectonic assemblages in the 4,000-km-long collisional orogeny; a-Zora blueschists, b-Tileouine/Tideridjaoine eclogites, c-Tin Essako, d-Égeré eclogite, e-Aleksod, f-Azorou N’Fad, g-Tin Begane, h-Gourma UHP eclogite, i-Assongo eclogite/blueschists, j-Kabyé Massif, k-Djabatouré Massif, l-Lato UHP eclogite, m-Akuze Massif, n-Forquilha retroeclogites, o-Central Brazil. Solid black stars indicate location of samples from this study (scale bar, 500 km). (c) Temporal distribution of the main lithotectonic units along each sector of the orogen together with main global events. Sr-isotope values for seawater after ref.17and pO2after ref.18. Timing of pre-collision geological events is mostly based on refs22,23,24,25,26,27,28. Figure 1: Geological context and tectonics of the West Gondwana Orogen. ( a ) Main cratons and tectonic blocks involved in the formation of the collisional West Gondwana Orogen (scale bar, 1,000 km). ( b ) Spatial distribution of high-pressure and ultrahigh-pressure rocks and main lithotectonic assemblages in the 4,000-km-long collisional orogeny; a-Zora blueschists, b-Tileouine/Tideridjaoine eclogites, c-Tin Essako, d-Égeré eclogite, e-Aleksod, f-Azorou N’Fad, g-Tin Begane, h-Gourma UHP eclogite, i-Assongo eclogite/blueschists, j-Kabyé Massif, k-Djabatouré Massif, l-Lato UHP eclogite, m-Akuze Massif, n-Forquilha retroeclogites, o-Central Brazil. Solid black stars indicate location of samples from this study (scale bar, 500 km). ( c ) Temporal distribution of the main lithotectonic units along each sector of the orogen together with main global events. Sr-isotope values for seawater after ref. 17 and pO 2 after ref. 18 . Timing of pre-collision geological events is mostly based on refs 22 , 23 , 24 , 25 , 26 , 27 , 28 . Full size image Deep subduction in the West Gondwana Orogen One main characteristic of the WGO is the existence of several mafic-ultramafic massifs containing relics of HP/UHP metamorphism [7] , [31] , [32] , [33] , [34] ( Fig. 1 ). To constrain the geochronological and petrological record of HP and UHP rocks across the WGO, we investigated eclogitic samples from Mali (S-506), Togo (DKE-350) and NE-Brazil (DKE-107) using coupled U-Th-Pb and rare earth element zircon analyses together with thermobarometric constrains. Eclogites from Mali and Togo are interlayered with HP/UHP quartzites from passive margin deposits [7] , [31] . They show a well-preserved peak paragenesis of garnet, omphacite, phengite, coesite/quartz and accessory rutile ( Fig. 2 ). Thermobarometric calculations for the peak eclogitic conditions were performed using a set of pressure sensitive net-transfer equilibria coupled with Fe-Mg exchange thermometry for the assemblage omphacite-garnet-phengite [35] combined with Zr-in-rutile [36] and Ti-in-zircon [37] thermometers ( Fig. 3 and Supplementary data 1 and 2 ). For the trace element thermometers, the activities of Zr or Ti and Si are fully buffered by the presence of rutile, zircon and quartz/coesite in all investigated samples. To calculate the peak-pressure conditions, we selected phases with petrographic evidence of equilibrium among omphacite with the highest jadeite content, garnet with the highest grossular and pyrope contents, and phengite with the highest Si content, as proposed by ref. 35 . Uncertainties given are according to the method followed in the study of each thermometer or barometer [35] , [36] , [37] . 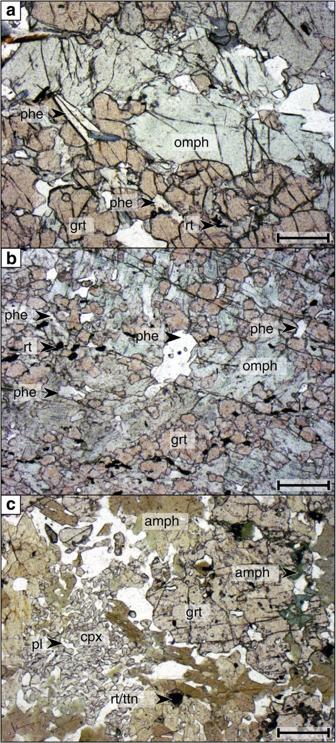Figure 2: Photomicrographs of the investigated samples. Eclogites from Mali (a) and Togo (b) exhibit phase equilibria among garnet (grt), omphacite (omph), phengite (phe) and rutile (rt) (scale bar, 500 μm). Retrogressed eclogites from NE-Brazil (c) have abundant amphibole (amph), garnet and clinopyroxene (cpx)+plagioclase (pl) symplectite after omphacite. In this sample rutile is commonly rimmed by titanite (ttn) (scale bar, 500 μm). Figure 2: Photomicrographs of the investigated samples. Eclogites from Mali ( a ) and Togo ( b ) exhibit phase equilibria among garnet (grt), omphacite (omph), phengite (phe) and rutile (rt) (scale bar, 500 μm). Retrogressed eclogites from NE-Brazil ( c ) have abundant amphibole (amph), garnet and clinopyroxene (cpx)+plagioclase (pl) symplectite after omphacite. In this sample rutile is commonly rimmed by titanite (ttn) (scale bar, 500 μm). 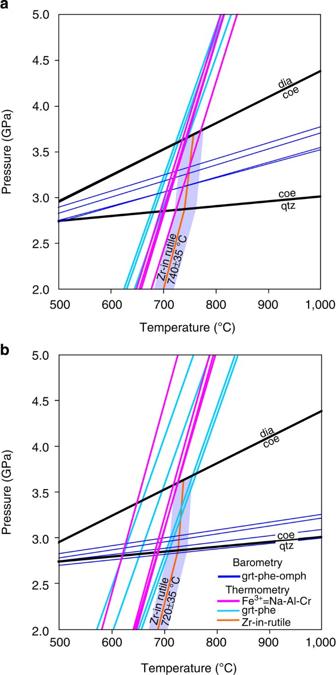Figure 3: Calculated equilibria for the ultra-high pressure rocks. (a) For the Mali (sample S-514) and (b) for Togo (sample DKE350) using the geothermobarometry of ref.35and the mineral composition data presented inSupplementary Data 1. Temperatures calculated with the garnet-phengite exchange reaction after ref.68and the Zr-in-rutile thermometer36using the data presented inSupplementary Data 2are also shown. The area in the diagram where the different barometer and thermometer intersect defines the P–T conditions of the mineral assemblage. Full size image Figure 3: Calculated equilibria for the ultra-high pressure rocks. ( a ) For the Mali (sample S-514) and ( b ) for Togo (sample DKE350) using the geothermobarometry of ref. 35 and the mineral composition data presented in Supplementary Data 1 . Temperatures calculated with the garnet-phengite exchange reaction after ref. 68 and the Zr-in-rutile thermometer [36] using the data presented in Supplementary Data 2 are also shown. The area in the diagram where the different barometer and thermometer intersect defines the P–T conditions of the mineral assemblage. Full size image Peak P-T condition in the Gourma region (Mali) was retrieved from an omphacite-garnet-phengite quartzite (sample S-514), which occurs in contact with the eclogites. Thermobarometric calculations using omphacite-garnet-phengite yielded a P-T range of 3.0–3.3 GPa (±0.3 GPa) and 690–705 °C (±65 °C) ( Fig. 3 ). Metamorphic zircons in the UHP Mali eclogite have 6–26 p.p.m. Ti, corresponding to Ti-in-zircon temperatures of 700–830 °C with a mean temperature of 720±20 °C in concordance with a mean Zr-in-rutile temperature of 740±35 °C. These metamorphic conditions are consistent with the rare occurrence of coesite-bearing eclogites and testify UHP conditions for this area, indicating subduction of the Gourma passive margin to depths of >100 km (ref. 6 ). Further south, in the Dahomey segment (Togo), UHP and HP eclogitic and granulitic rocks are exposed in the Lato region [31] . For the Togo eclogite, calculations indicate P-T conditions in the range of 2.8–3.0 GPa (±0.3 GPa) and 620–700 °C (±65 °C) ( Fig. 3 ). Ti-in-zircon temperatures range from 640 to 760 °C with a mean temperature of 680±20 °C, which is in agreement with the mean temperature of Zr-in-rutile of 720±30 °C. Although no coesite relics have been found so far in Togo, calculated P-T conditions are well within the coesite stability field, suggesting UHP metamorphism. Eclogites from NE-Brazil are found as boudins within high-temperature, partially melted metasedimentary rocks [32] . As a consequence, they are intensely retrogressed and composed of garnet, Ca-rich pyroxene, hornblende and symplectite of Na-augite and plagioclase. From the composition of relic phases, minimum P-T conditions for the decompression stage of 1.7 GPa and 770 °C have been established [32] . In the investigated sample DKE-107, zircon displays striking similarities in age and composition to the zircon retrieved from the UHP rocks, but thermobarometric or mineralogical evidence for UHP conditions is yet to be demonstrated. Ti-in-zircon temperatures yield a mean temperature of 700±15 °C for type-1 and 690±15 °C for type-2 zircons (see below). The mean Zr-in-rutile temperatures of 790±35 °C are slightly higher than those recorded by Ti-in-zircon, potentially recording increasing temperature during decompression from the eclogite to the granulitic stage. In Hoggar (Algeria), the c. 620 Myr Tideridjaouime-Tileouine-Tassendjanet HP metamorphic units (550–650 °C, 1.4–2.2 GPa) represent a slab of subducted continental material that is now exposed along the edge of the IOGU terrane, which has been interpreted as a microcontinent [34] , [38] . In the southern LATEA terrane, the Tin Begane eclogite (790 °C, 1.5 GPa) is preserved as boudins within the thrust zone of an allochthonous supracrustal sequence [39] . The Azroun N’Fad eclogite represents the deepest unit within the LATEA terrane owing to the highest pyrope content of relict garnet (up to 44%), with a decompression path from 1.5 to 1.1 GPa between 800 and 700 °C (ref. 40 ). Timing of deep continental subduction The HP/UHP samples investigated contain zircons that were imaged by cathodoluminescence to show internal zoning, dated by the U-Pb method with a Sensitive High Resolution Ion Microprobe (SHRIMP) and characterized for their trace element composition by Laser Ablation Inductively Coupled Plasma Mass Spectrometer (LA-ICP-MS) (See Methods below). The zircon crystals from the Mali and Togo eclogite are composed of relict cores and metamorphic rims and minor rounded homogeneous zircons. The cores show regular zoning ( Fig. 4 ) and high Th/U (0.5–0.4) and rare earth element (REE) contents. The zircon REE pattern is enriched in heavy-REE (HREE) and shows a marked negative Eu anomaly ( Fig. 4 ). All these features are consistent with a magmatic origin [41] . The zircon cores from the Mali eclogite are severely discordant and yield spurious individual ages ( Supplementary Data 3 ), which suggest partial resetting of the U-Pb system. An upper discordia intercept points to a protolith age of >1.0 Ga. For the Togo eclogite, the zircon cores yield a protolith age of 703.2±8.1 Myr. 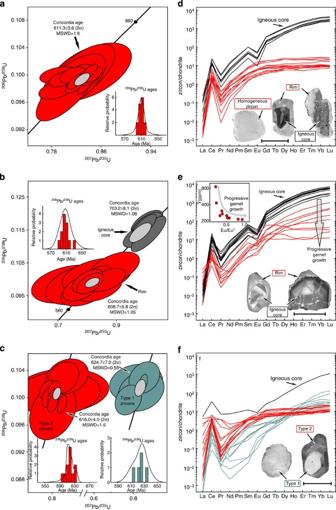Figure 4: Zircon geochronology and trace elements. Wetherill Concordia plots of U-Pb zircon data from (a) Gourma region, Mali (sample S-506); (b) Lato region, Togo (sample DKE-350); (c) Forquilha region, NE-Brazil (sample DKE-107). Ellipse colours reflect zircon growth domains as defined by zoning and REE composition. The light grey ellipse at the centre of data cluster represents the Concordia age. The probability density diagram of206Pb/238U ages in each cluster is shown as an inset. Internal structure of the zircons (scale bar, 80 μm) revealed by cathodoluminescence and rare earth element (REE) composition (chondrite-normalised patterns) for each zircon type for (d) Gourma region, Mali (sample S-506); (e) Lato region, Togo (sample DKE-350); (f) Forquilha region, NE-Brazil (sample DKE-107). Inset ineillustrates the combined decreasing of Y and negative Eu anomaly, indicating growing of zircon rim with increasing garnet modal abundance in the Lato eclogite (sample DKE-350). Figure 4: Zircon geochronology and trace elements. Wetherill Concordia plots of U-Pb zircon data from ( a ) Gourma region, Mali (sample S-506); ( b ) Lato region, Togo (sample DKE-350); ( c ) Forquilha region, NE-Brazil (sample DKE-107). Ellipse colours reflect zircon growth domains as defined by zoning and REE composition. The light grey ellipse at the centre of data cluster represents the Concordia age. The probability density diagram of 206 Pb/ 238 U ages in each cluster is shown as an inset. Internal structure of the zircons (scale bar, 80 μm) revealed by cathodoluminescence and rare earth element (REE) composition (chondrite-normalised patterns) for each zircon type for ( d ) Gourma region, Mali (sample S-506); ( e ) Lato region, Togo (sample DKE-350); ( f ) Forquilha region, NE-Brazil (sample DKE-107). Inset in e illustrates the combined decreasing of Y and negative Eu anomaly, indicating growing of zircon rim with increasing garnet modal abundance in the Lato eclogite (sample DKE-350). Full size image The zircon rims in the Mali and Togo eclogite show a distinct internal texture, chemistry and age. They have weak or no zoning, low REE contents with flat HREE patterns in the Mali sample and steep to flat HREE patterns in the Togo sample. In contrast to the cores, the zircon rims commonly have lower Th/U (mostly 0.01–0.09) and no significant Eu anomaly. Depletion of HREE together with the lack of negative Eu anomaly indicates that these zircons have grown in the presence of garnet and in the absence of plagioclase [41] . This mineral assemblage is diagnostic of eclogite-facies conditions. For the Togo zircons, the decreasing HREE+Y content ( Fig. 4 inset) is consistent with zircon rim growth over a period with increasing garnet modal abundance, as expected during prograde metamorphism. For the Mali samples, 15 analyses yield a concordia age of 611.3±3.6 Myr, and for the Togo samples the rims are dated at 608.7±5.8 Myr ( Fig. 4 ). As individual zircon domains that grew during prograde to peak metamorphism in the Togo sample show no age difference within the analytical resolution (c. 12 m.y. ), a rapid tectonic burial rate can be inferred for the Togo eclogite. Zircons from the NE-Brazil eclogite have rare magmatic cores and two distinct metamorphic domains. The texturally older metamorphic domain is U-poor, commonly rounded and displays no internal structure (type 1 in Fig. 4 ). The texturally younger, U-richer domain shows weak or no zoning (type 2). Type 1 zircons are HREE-enriched and middle-REE-depleted when compared with the type 2 zircons, which have a flat HREE pattern with no negative Eu anomaly, similar to the eclogite-facies zircon rims from Togo and Mali. Changes in REE pattern between types 1 and 2 are attributed to middle-REE-rich titanite breaking down to rutile and increasing garnet growth during burial to HP conditions. The two chemically different zircon domains yield ages that are within error, but support their textural relationships: the inner, U-poor rims are 624.7±7.0 Myr ( n =5, 2-sigma) while the outer rim is dated at 616.0±4.0 Myr. The P-T determinations for the Mali and Togo samples provide evidence for subduction of a continental margin to UHP conditions ( Fig. 5 ). The metamorphic zircon domains in the HP/UHP rocks from Mali, Togo and NE-Brazil have a trace element composition, indicating growth at high-pressure conditions (flat HREE pattern and no negative Eu anomaly). In the Togo and NE-Brazil samples, zircon growth also occurred during prograde metamorphism and burial. The ages for eclogite-facies metamorphism in Mali (611±6 Myr, forced to 1% to account for external errors), Togo (609±6 Myr) and NE-Brazil (616±6 Myr) indicate synchronous subduction (within the resolution of the technique) in these localities of the WGO. In Hoggar, the age for high-pressure metamorphism partially overlaps with the results from eclogites investigated in this study (623±6 Myr (ref. 34 )), suggesting that HP/UHP metamorphism and continental subduction extended over at least 2,500 km along the WGO within a time window of <20 Myr. ( Fig. 5 ). This is a unique scenario in the Ediacaran Earth and represents a continental collision front that is comparable in size to the modern Himalaya ( Fig. 1 ). 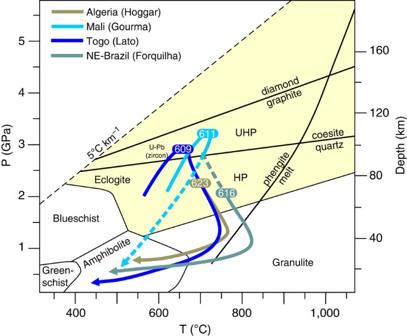Figure 5: Pressure-temperature paths for the high-pressure and ultrahigh-pressure terranes from West Gondwana Orogen. Peak metamorphic conditions for Mali and Togo eclogites are discussed in the text and data are available in the electronic appendix (dashed curves are inferred). In the Algerian sample, the peak eclogitic stage (2.2–2.0 GPa and 650 °C)34was followed by a post peak heating and exhumation at 1.4–1.0 GPa and 730 °C (ref.34) and cooling at 1.0–0.7 GPa and 610 °C (ref.34). No geothermobarometric information is available for the retrograde P-T path in Mali, but petrographic6and geochronological7evidence suggests rapid exhumation without passing through the granulite field. Previous geothermobarometric data from Lato terrane, Togo, indicate a retrograde path through granulite-facies (1.0–0.8 GPa and 700–750 °C)31and later amphibolite-facies (0.6–0.4 GPa and 500–600 °C)31. Minimum calculated P-T condition for the NE-Brazil retrogressed eclogites are 1.7 GPa and 770 °C (ref.32); this was followed by a granulitic stage (1.4 GPa and 870 °C) and then an amphibolitic stage (0.5–0.75 GPa and 530–700 °C)32. Figure 5: Pressure-temperature paths for the high-pressure and ultrahigh-pressure terranes from West Gondwana Orogen. Peak metamorphic conditions for Mali and Togo eclogites are discussed in the text and data are available in the electronic appendix (dashed curves are inferred). In the Algerian sample, the peak eclogitic stage (2.2–2.0 GPa and 650 °C) [34] was followed by a post peak heating and exhumation at 1.4–1.0 GPa and 730 °C (ref. 34 ) and cooling at 1.0–0.7 GPa and 610 °C (ref. 34 ). No geothermobarometric information is available for the retrograde P-T path in Mali, but petrographic [6] and geochronological [7] evidence suggests rapid exhumation without passing through the granulite field. Previous geothermobarometric data from Lato terrane, Togo, indicate a retrograde path through granulite-facies (1.0–0.8 GPa and 700–750 °C) [31] and later amphibolite-facies (0.6–0.4 GPa and 500–600 °C) [31] . Minimum calculated P-T condition for the NE-Brazil retrogressed eclogites are 1.7 GPa and 770 °C (ref. 32 ); this was followed by a granulitic stage (1.4 GPa and 870 °C) and then an amphibolitic stage (0.5–0.75 GPa and 530–700 °C) [32] . Full size image On the basis of the oldest known UHP rocks in Mali [7] , it has been proposed that this time marks the onset of modern plate tectonics [14] , [15] . There is a general consensus that continent–continent collisional settings ultimately create high topography. Deep subduction of felsic continental crust leads to collisional zones with deep roots that consist of material with a density lower than mantle rocks [3] , [42] . This density contrast produces an isostatic rebound that gives rise to significant topographic relief [43] , [44] . Combined with stacking and flow of crustal units during the thickening and exhumation, this continent–continent type collision may have produced mountains with higher average altitudes than pre-Neoproterozoic orogens had and where UHP rocks are not found. Indeed, most UHP rocks are exposed within large mountain belts like the present Alps and the Himalayas or the now-eroded Paleozoic orogens [3] . Therefore, the finding of rocks that underwent relatively low temperatures and HP to UHP conditions in a continental collisional setting is a tracer not only for paleo-subduction zones (sutures) but also for large mountain edifices. Maximum elevation would have been constrained by the limits of crustal strength [11] and also by the extent of high mountain glaciation through an efficient denudation mechanism known as the ‘glacial buzzsaw’ [45] . Relief is a primary regulator of erosion rate as documented in present mountain belts and supported by recent modelling [46] . In the Alps, the rise of the mountains is related to the continental collision, immediately following the subduction of the European continental margin at c. 35 Myr (refs 1 , 2 , 3 , 4 ). In the Himalayas, UHP metamorphism and deep continental subduction is dated at c. 50 Myr (ref. 47 ). Stable isotope paleoaltimetry shows that central Tibet has been at an elevation similar to its modern elevation since c. 40–26 Myr (refs 48 , 49 ), providing evidence that a high relief can be sustained for at least 40 Myr postdating subduction of the continental margin. In the Himalayan collisional orogen, 4- to 5-km-thick deltaic sediments extending over 3,000 km into the Indian Ocean were deposited over the last 7 m.y., in the late-stage exhumation of the orogen [50] . We propose that a high-altitude mountain range existed in the WGO in the period 620–570 Myr and was, therefore, a likely source for vast amounts of erosional sediments. The sink for the detritus related to the dissection of the WGO collisional chain is preserved within post-collisional foreland basins, or remnant Ediacaran seaways ( Fig. 1 ), usually to the west of the orogen. The best examples are the Gourma and Taoudeni basins [51] in Algeria and Mali, the upper portion of the Volta Basin [52] in Togo and Ghana, and the Paraguay and Bambuí basins in Central Brazil where Ediacaran biota have been described [53] , [54] . The Ediacaran sedimentary rocks in South America are partially masked by younger sedimentary cover; evidence from the Parecis basin in the southwestern portion of the Amazon craton indicates that the extent of the Ediacaran forelands could be larger than previously thought [55] . The high mountain relief produced as a result of the Himalayan-scale continental subduction and collision along the WGO in the Late Ediacaran (620–610 Myr) has the appropriate time to shed sediments vital to the rise of the metazoans at c. 600–575 Myr (the so-called Ediacaran Fauna). A number of authors have recognized that nutrients such as P, Ca, K, Fe, Mg, Zn and Mo from continental sediments are essential to sustain complex life forms [56] . Ediacaran life radiation was also aided by increased oxygen in the atmosphere and oceans [18] . It has been proposed that the environmental conditions suitable for life radiation were strongly influenced by high and rapidly increasing rates of sediment accumulation and subsidence associated with amalgamation of the Gondwana supercontinent [57] . The systematic increase in 87 Sr/ 86 Sr ratios in the seawater during Ediacaran period reflects the addition of soluble Sr derived from erosion of old continents into oceans [18] . Erosion of mountains that were produced during the amalgamation of supercontinents has also been linked to steep rises in atmospheric O 2 (refs 19 , 21 ), as it provided nutrients for algae and cyanobacteria responsible for the photosynthetic production of O 2 . Increased sedimentation and burial of organic carbon and pyrite [21] prevents their reaction with oxygen in the environment, leading to further increases in atmospheric oxygen. While there is strong evidence for a link between erosion, nutrient supply and increased biological activity, further research is needed to fully quantify fluxes and bioavailability of critical elements. Previous geochronology of zircons from sediments has suggested that the erosion of the Transgondwana supermountains that formed at the collision of East and West Gondwana [20] was responsible for the supply of nutrients necessary for life radiation. However, the timing is problematic as this poly-phased orogen was completely assembled only at c. 520–500 Myr (ref. 58 ), and therefore post-dates the Ediacaran life radiation. The Ediacaran organisms first appeared in interglacial and post-glacial environments between 600 and 560 Myr and later colonized environments around the world in a variety of facies, in both shallow and deep water showing little geographic endemism [16] . Our rationale is also consistent with the view that the ancestries of the larger Cambrian explosion, which includes the Ediacaran metazoans, extend some 50–70 million years before its expression in the fossil record [59] , thus placing the WGO as one of the potential environmental triggers for life sustainability on the planet. We report the timing and significant extent of the oldest known deep continental subduction in geological history, which makes the West Gondwana Orogen one of the events that could have changed the way evolution proceeded on Earth. Mineral chemistry Chemical analyses of major elements in minerals ( Supplementary Data 1 ) were performed on polished thin sections with a CAMECA SX100 electron microprobe at the Research School of Earth Sciences (RSES), Australian National University (ANU), operating in the wavelength-dispersive mode. Acceleration voltage and beam current were 15 kV and 20 nA with a beam diameter of 1μm for pyroxene and garnet and 5 μm for micas. Counting times per element were 20 s for Na, Mg, Si, Al, K, Ca and Fe and 60 s for Ti, Cr and Mn. K and Na were always analysed first in the routine. Several analyses on each phase were performed to obtain representative compositions, and core-rim analyses were done to assess zoning patterns. Standards were natural and synthetic minerals, which were all determined on the Kα emission peak. In-house mineral standards were used as secondary standards. Imaging of internal zoning Zircons were separated from the crushed rocks using conventional heavy liquid and magnetic techniques. Grains were mounted in epoxy resin and polished down to expose the near-equatorial section. Imaging of grain sections was carried out at the RSES in Canberra and at the Geochronological Research Centre (CPGeo), the University of São Paulo (USP). Cathodoluminescence (CL) investigation at RSES used a JEOL-6610 A scanning electron microscope (SEM) supplied with a Robinson detector for cathodoluminescence. Operating conditions for the SEM were 15 kV, 70 μA and a 20 mm working distance. In Sao Paulo, CL images were acquired using a Quanta 250 FEG SEM equipped with a Centaurus Mono CL3+ detector for cathodoluminescence. Trace elements Trace elements of zircon and rutile ( Supplementary Data 2,3 ) were analysed by laser-ablation inductively coupled plasma mass spectrometry (LA-ICP-MS) at the RSES, ANU, as reported in ref. 60 . The instrument includes an ANU ‘HelEx’ laser ablation cell built to receive a pulsed 193 nm wavelength ArF Excimer laser with 100 mJ output energy at a repetition rate of 5 Hz and coupled to an Agilent 7500, s quadrupole ICPMS. The instrument was tuned for maximum sensitivity and minimum production of molecular species, maintaining ThO + /Th + at <0.5%. The laser was operated in drilling mode with spot sizes of 47 μm for rutile and 28 μm for zircon. Total analysis time was ~60 s, the first ~25 s of which was background acquisition before ablation. Synthetic glasses (NIST 612 for zircon and NIST 610 for rutile) were used for external calibration and values were taken from ref. 61 . Internal standards were SiO 2 of 32.45 wt% for zircon and TiO 2 of 98 wt% for rutile. The BCR-2 G natural glass was used as a secondary standard to monitor accuracy. Data evaluation was done with the software package Iolite v.2.5 . Chondrite values for normalization are from ref. 62 . Sensitive high resolution ion micro probe Zircon was analysed for U, Th and Pb in the epoxy mount using the SHRIMP-II at the RSES at ANU in Canberra and the SHRIMP-IIe at USP in São Paulo. For zircon, instrumental conditions and data acquisition were generally as described previously [63] . The data were collected in sets of six scans throughout the masses, and a reference zircon (TEMORA [64] ) was analysed each fourth analysis. The analyses ( Supplementary Data 4 ) were corrected for common Pb on the basis of the measured 207 Pb/ 206 Pb ratios as described previously [63] . The common Pb composition was assumed to be that predicted by the model of ref. 65 . U-Pb data were collected over five analytical sessions using the same standard, with the different sessions having calibration errors between 1.23% and 2.16% (2 sigma), which was propagated to single analyses. Data evaluation and age calculation were done using the software Squid and Isoplot/Ex, respectively [66] , [67] . Average 206 Pb/ 238 U ages are quoted at the 2-sigma confidence level and forced to at least 1% to account for external errors. How to cite this article : Ganade de Araujo, C. E. et al. Ediacaran 2,500-km-long synchronous deep continental subduction in the West Gondwana Orogen. Nat. Commun. 5:5198 doi: 10.1038/ncomms6198 (2014).